Catalytic asymmetric C–Si bond activation via torsional strain-promoted Rh-catalyzed aryl-Narasaka acylation Atropisomers are important organic frameworks in bioactive natural products, drugs as well as chiral catalysts. Meanwhile, silanols display unique properties compared to their alcohol analogs, however, the catalytic synthesis of atropisomers bearing silanol groups is challenging. Here, we show a rhodium-catalyzed torsional strain-promoted asymmetric ring-opening reaction for the synthesis of α-silyl biaryl atropisomers. The reaction features a dynamic kinetic resolution of C(Ar)-Si bond cleavage, whose stereochemistry was controlled by a phosphoramidite ligand derived from ( S )-3-methyl-1-((2,4,6-triisopropylphenyl)sulfonyl)piperazine. This work is a demonstration of an aryl-Narasaka acylation, where the C(Ar)-Si bond cleavage is promoted by the torsional strain of α, α’-disubstituted silafluorene. Atropisomers are an important class of compounds, which showcased chirality due to the restricted rotation around the single C–C, C–N, or C–O bonds [1] , [2] , [3] . Among them axially chiral biaryls have caught extensive attentions due to their wide existence in bioactive natural products, drugs [4] , [5] ; furthermore it is one of prior skeletons for chiral ligands or catalysts in asymmetric catalysis. Despite the importance of biaryl atropisomers, the catalytically asymmetric synthesis was challenging due to the steric hindrance around the axis, which usually required three or four ortho substituents for achieving stable axial chirality [6] . The aryl–aryl cross-coupling or oxidative coupling is the most straightforward method, which delivered extremely useful axially chiral ligands and catalysts, such as BINOLs [7] , [8] , [9] , [10] , [11] , [12] , [13] , [14] , [15] , [16] , [17] , [18] . In addition, other useful methods, including (dynamic) kinetic resolution [19] , [20] , [21] , [22] , [23] , [24] , [25] , [26] , point to axial chirality transfer [27] , [28] , [29] , de novo aryl ring synthesis [30] , [31] , [32] , [33] , [34] have been developed and significantly broadened the diversity of biaryl atropisomers. Recently, organo-catalyzed transformation showed its strong power in organic synthesis and it have been successfully applied to axially chiral molecules construction [35] , [36] , [37] , [38] , [39] , [40] . In comparison with the classic asymmetric couplings, which proceed via a highly bulky metal intermediate (Fig. 1a ), the ring-opening strategy surcumvented this key intermediate and it provided an efficient protocol for construction of biaryl atropisomers. Bringmann pioneered the atropisomer synthesis via ring-opening of lactones, with either stoichiometric or catalytic methods (Fig. 1b ) [41] , [42] . Recently, Zhang and co-workers realized Ir-catalyzed asymmetric hydrogenation of Bringmann’s lactones [43] . Under the catalysis of nickel, copper, and palladium, the groups of Hayashi, Gu and others realized the ring-opening of dibenzo[b,d]thiophenes [44] , diaryliodoniums [45] , [46] , [47] , [48] , and 9 H -fluoren-9-ols (Fig. 1b ) [49] . This ring-opening reactions showed particular advantages in the preparation of sterically hindered ortho tetra-substituted atropisomeric biaryls; furthermore, these ring-opening reactions displayed excellent diversity: hydroxyl, hydroxymethyl, thiol, iodine, and keto groups were efficiently introduced to the position adjacent to the chiral axis. Fig. 1: Ring-opening strategies for atropisomer synthesis. a Asymmetric aryl–aryl cross-coupling. b Ring-opening strategy for the construction of axially chiral biaryls. Full size image Silanols display unique applications in pharmaceutical chemistry and organic chemistry [50] , [51] . For example, compound 1 displays nuclear receptor modulator activity and has better lipophilicity than the corresponding carbinol [52] . Silanols 2 and 3 were used as organocatalysts for asymmetric syntheses [53] , [54] . Considering the remarkable property of silanol groups, we wonder if ortho silanol substituted biaryl atropiosmers could be accessed via the carbon–silica bond cleavage of silafluorene in a stereoselective manner. Unfortunately, the silanes showed low reactivity in classic cross-couplings, i.e., Hiyama or Hiyama–Denmark Couplings [55] , [56] . Pleasingly, the Narasaka acylation [57] , [58] , which favored C–SiMe 3 bond breaking over the C–SiMe 2 (OH), provided a potential solution for C–Si bond cleavage of silafluorene (Fig. 2b ). However, challenges still remain: (a) only vinyl silanes underwent Narasaka acylation; (b) it is necessary to differentiate up to four C(aryl)–Si bonds in our systems. The releasing of noncyclic aryl ring is the undesired pathway; (c) the classic Narasaka acylation is steric sensitive, and vinyltriphenylsilane displayed extremely low reactivity (Fig. 2c ). It is forseeable, the reaction would be more challenging if tetra(arylsilanes) were used. In the previous studies on the ring-opening reactions, we found that the two non-hydrogen groups adjacent to the axis increased the distortion of the molecule. The distorted molecule is the energetic compound, which had relative lower activation energy than the non-distorted one for the ring-opening reaction. Different from the inherent high strain of three- or four-membered rings, we anticipated that the activity of ring-opening reaction can be increased by the torsional strain of α, α′-disubstituted five-membered silafluorenes. Furthermore, the torsional strain also enabled to differentiate one of four C(aryl)–Si bonds to give desired products. Fig. 2: Carbon–silica bond cleavage for atropisomer synthesis. a Silanols in drug scaffold or ligands. b Narasaka acylation and Hiyama coupling. c Asymmetric Narasaka acylation for atropisomer synthesis. Full size image Here, we report an aryl-Narasaka acylation reaction catalyzed by the chiral rhodium complex which is in situ formed of [Rh(CO) 2 Cl] 2 and phosphoramidite ligand derived from ( S )-3-methyl-1-((2,4,6-triisopropylphenyl)sulfonyl)piperazine. Computational studies show that the storioanl stain of 7,7-diphenyl-7 H -dinaphtho[2,1- b :1′,2′- d ]silole is about 12.58 kcal mol −1 , which efficiently accelerate the C–Si bond cleavage. 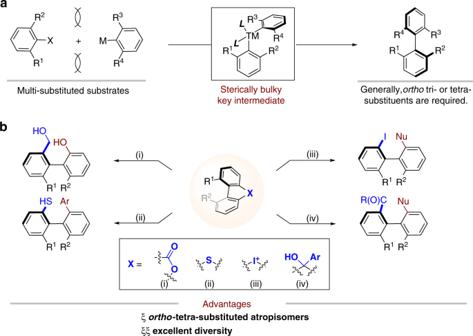Fig. 1: Ring-opening strategies for atropisomer synthesis. aAsymmetric aryl–aryl cross-coupling.bRing-opening strategy for the construction of axially chiral biaryls. Optimization of Rh-catalyzed aryl-Narasaka acylation Our investigation began with the ring-opening/acylation reaction of dimethyl silafluorene ( 4a ) [59] , [60] , [61] , [62] with acetic anhydride ( 5a ) (Table 1 ). With [Rh(CO) 2 Cl] 2 as the catalyst, primary investigations found that the TADDOL-based phosphoramidite L1 gave satisfied stereo-induction with 49% yield in the presence of 1.0 equiv of Cs 2 CO 3 (Table 1 , entry 1). Decreasing the loading of base gradually improve the yield of 6a , until it reached the highest level when 30 mol% of Cs 2 CO 3 was employed (Table 1 , entries 2–4). Surprisingly, the reaction without the addition of base did not produce isolable desired product (Table 1 , entry 5). Replacing the biphenyl group in the ligand with 4-fluorophenyl group gave a decreased enantioselectivity (Table 1 , entry 6). The ligand without the chiral α-methyl group at the piperidine moiety ( L3 ) afforded a reduced stereoselectivity (Table 1 , entry 7). Organic base, i.e., Et 3 N was not suitable for this ring-opening/acylation reaction, while Na 2 CO 3 dramatically improved the yield and maintained high enantioselectivity (Table 1 , entries 8–9). The additives, such as KBr or 4 Å molecular sieve did not offer better outcomes (Table 1 , entries 10–11). Table 1 Optimization of reaction conditions a . Full size table The synthesis of sterically hindered silanols is challenging [63] , [64] . Unfortunately, applying the optimized conditions ([Rh(CO) 2 Cl] 2 / L1 ) to 4a and benzoic anhydride gave conspicuously decreased ee value (54%, 75% ee). 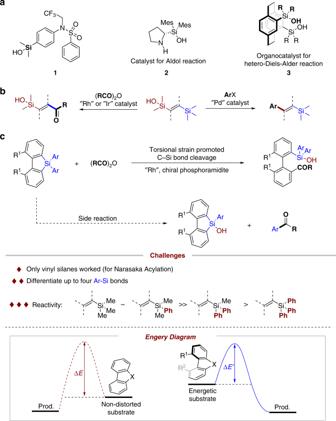Fig. 2: Carbon–silica bond cleavage for atropisomer synthesis. aSilanols in drug scaffold or ligands.bNarasaka acylation and Hiyama coupling.cAsymmetric Narasaka acylation for atropisomer synthesis. Thus, further optimization based on the modification of phosphoramidites were carried out by using Si , Si -diphenylsilafluorene 4b and benzoic anhydride (Table 2 ). The N -Cbz or N -Boc piperazine derived ligands L4 and L5 gave improved results in comparison with L1 (Table 2 , entries 1–3). The 2,4,6-trimethylphenylsulfonamide analog L6 gave 77% ee, while, pleasingly, 2,4,6-tri(isopropyl)phenylsulfonamide derivative L7 afforded the desired product 6b in 92% ee (Table 2 , entries 4 and 5). The use of Cs 2 CO 3 dramatically improved the yield (Table 2 , entry 6). Decreasing the loading of L7 to 6.25 mol% gave slightly lower yield of 4b (Table 2 , entry 7). Increasing the amount of Cs 2 CO 3 is detrimental for the yield (Table 2 , entries 8 and 9). Further optimization by using Et 3 N in lieu of Cs 2 CO 3 , or addition of molecular sieve did not produce better results (Table 2 , entries 10 and 11). Table 2 Re-optimization for diphenylsilafluorene a . Full size table Substrate scope Under the optimal conditions, a number of acid anhydrides were tested with 4b as the substrate (Fig. 3 ). The aliphatic anhydrides also smoothly coupled with 4b to produce the corresponding silonols. The longer alkyl chain slightly decreased the yields and selectivity ( 6c – 6f ). 2-Methoxyacetic anhydride steadily underwent this acylation reaction to give 6g in excellent yield and enantioselectivity. The reaction of cyclopropanecarboxylic anhydride afforded the product 6h in 81% yield with 85% ee. The acrylic anhydride derivatives also reacted with 4b uneventfully to furnish the products in excellent ee values ( 6i – 6k ). The aromatic anhydrides were also compatible substrates. The p -methylbenzoic anhydride gave a slightly decreased yield, while the electron-withdrawing substituents were advantageous for both yields and stereoselectivity ( 6l – 6o ). Subsequently, other substituted aromatic acid anhydrides, including 3,4,5-trimethoxybenzoic anhydride, were submitted to the standard conditions to produce the corresponding silanols 6p – 6s with excellent ees. Lastly, the 2-naphthoic or heteroaromatic anhydride were checked, and both of the reactions proceeded smoothly with the ee values were marginally changed ( 6t and 6u ). Fig. 3: Substrate scope a . a Reaction conditions: silafluorene 4b (0.20 mmol) and acid anhydrides (0.30 mmol, 1.5 equiv), [Rh(CO) 2 Cl] 2 (0.005 mmol, 2.5 mol%), L7 (0.0125 mmol, 6.25 mol%), and base (30 mol%, Na 2 CO 3 for aliphatic anhydride, Cs 2 CO 3 for aromatic anhydride) in 1,4-dioxane (4.0 mL) at 70 °C for 24 h. b L1 was used as the ligand. c The reaction time is 48 h. Full size image Silafluorenes bearing different substituents were further investigated (Fig. 4 ). Ligand L1 was found more efficient for substrate 4a , which reacted with propionic anhydride and butyric anhydride to give 6v and 6w in 85% and 90% ee, respectively. The substituted benzene rings attached to the silicon atom have marginal effect on the selectivity, all the silanols were formed in excellent stereoselectivity ( 6x – 6bb ). The silafluorenes with biphenyl skeleton gave relatively lower stereoselectivity ( 6cc – 6ee ). The diastereochemistry of compound 6cc was determined to be R by single crystal X-ray diffraction analysis (CCDC 1968743). The starting material α,α′,β,β′-tetramethyl biphenylsilafluorene showed slight poor stability, as a result, the corresponding product 6ff was isolated in only 45% yield with 87% ee. Fig. 4: Substrate scope a . a Reaction conditions: silafluorene 4 (0.20 mmol) and acid anhydride 5 (0.30 mmol, 1.5 equiv), [Rh(CO) 2 Cl] 2 (0.005 mmol, 2.5 mol%), L7 (0.021 mmol, 10.5 mol%) and base (30 mol%, Na 2 CO 3 for aliphatic anhydride, Cs 2 CO 3 for aromatic anhydride) in 1,4-dioxane (4.0 mL) at 70 °C for 24 h. b The reaction was performed with L1 as the ligand at 50 °C for 48 h. Full size image Control experiments For the unsymmetrical silafluorene 4j , the reaction gave 1:1 diastereomers, although both 6gg (CCDC 2013379) and 6gg′ were obtained in high enantioselectivity (Fig. 5a , eq (1)). The reaction between 4b and benzoic 4-fluorobenzoic anhydride afforded 6m and 6b in a ratio of 1:1.3 (Fig. 5a , eq (2)). Notably, with acetic benzoic anhydride as the reagent, the reaction produced methyl aryl ketone 6c as the major product ( 6c : 6b = 6.7:1) (Fig. 5a , eq (3)). Finally, a control reaction by mixing 4a and 4b (1:1) was performed with acetic anhydride as limiting reagent. It afforded a 1.5:1 mixture of 6a and 6c , indicating 4a was slightly more active than 4b under our conditions (Fig. 5b , eq (4)). Fig. 5: Selectivity for unsymmetrical substrates and synthetic applications. a Reactions of nonsymmetric substrates. b Reactivity of different substituted substrates using acetic anhydride as limiting reagent. c Synthetic application of axially chiral silanols. Full size image Synthetic application Treatment of 6b with phenylmagnesium chloride at 0 °C afforded hydroxysilanol 7 in excellent yield (Fig. 5c , eq (5)). Compound 7 was an anologue of corresponding carbols, which was potentially useful in asymmetric catalysis, for example, asymmetric hetero-Diels–Alder reactions [65] . In addition, vinylation of the ketone, followed by bromocyclization gave cyclic compound 9 (CCDC 1987455) in excellent diastereoselectivity (Fig. 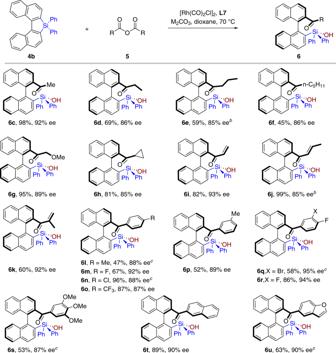Fig. 3: Substrate scopea. aReaction conditions: silafluorene4b(0.20 mmol) and acid anhydrides (0.30 mmol, 1.5 equiv), [Rh(CO)2Cl]2(0.005 mmol, 2.5 mol%),L7(0.0125 mmol, 6.25 mol%), and base (30 mol%, Na2CO3for aliphatic anhydride, Cs2CO3for aromatic anhydride) in 1,4-dioxane (4.0 mL) at 70 °C for 24 h.bL1was used as the ligand.cThe reaction time is 48 h. 5c , eq (6), (7)) (For reaction conditions optimization, see Supplementary Table 1 ). The Hiyama coupling by employing these silanols was not successful under various conditions, which was possibly due to the steric hindrance of the silanols. However, silanol 6b was readily transferred to arylbromide 10 , which underwent classic cross-coupling to give 11 without losing the enantiopurity (Fig. 5c , eq (8)). Mechanistic studies For comparison, compound 4c was also synthesized, and notably silanol 4c showed poor reactivity under standard conditions. To get some structural information of these silafluorenes, single crystals of both 4a (CCDC 1968747) and 4c (CCDC 1968985) were obtained and analyzed by X-ray diffraction. It clearly shows the biphenyl structure in 4c is almost planar, while the increased size of compound 4a makes the naphthyl rings no longer coplanar. It is a twisted molecule with a distortional angle being 31.8° of the binaphthyl skeleton (Fig. 6a ). We calculated the rotational barrier [Δ G g (298.15 K, 1 atm) ] of 4a , which is around 20.4 kcal/mol. Thus, the calculated half-life of 4a is around 94 s at room temperature (Fig. 6b ). In order to learn more about the torsional strain energy of 4a , we calculated the hydrogenation energies of 4a and 4c , respectively (Fig. 6c ). Considering the structural differences between 4a and 4c , we further calculated the hydrogenation energy of noncyclic compounds 4a′ and 4c′ (for details see Supplementary Table 2 ). Thus, the torsional strain energy of 4a is calculated as below: 
    ΔG_g (298.15  K,   1  atm) 	= (ΔG1 - ΔG2) - (ΔG1^' - ΔG2^')
     	= 12.58  kcal  mol^-1. Fig. 6: Structure and activity relationship. a Relationship between structure and reactivity of silafluorene. b calculated rotational barrier energy of 4a . c Calculated torsional strain energy of 4a . d Preparation of Rhodium-ligand complex. Full size image Markedly, the treatment of [Rh(CO) 2 Cl] 2 with one molar ratio of phosphoramidite L7 in dichloromethane formed a yellowish dimer [Rh(CO)Cl( L7 )] 2 by releasing two molecules of CO. Recrystallization of this complex in ethyl acetate/hexanes gave a reddish orange crystal that was suitable for X-ray crystallography analysis (CCDC 1969002) (Fig. 6d ). In this crystal structure, the (2,4,6-triisopropylphenyl)sulfonylpiperazine moiety worked as a large group by shielding one face of the rhodium center. Based on the above results and previous studies on Narasaka acylation [66] , a brief catalytic cycle was tentitatively proposed (Fig. 7 ). The coordination of L7 to the pre-catalyst formed monomer Rh(I) complex. The oxidative addition of Rh(I) with silafluorene 4b cleavaged C(Ar)–Si bond to form 10 , which gave optically active biaryl intermediate 11 via reductive elimination forming a Si–O bond. Subsequently, the second oxidation between 11 with acid anhydride 5 delivered Rh(III) complex 12 . Reductive elimination of 12 furnished acylation product 13 , which would give the final product 6 after hydrolysis of tri(aryl)silyl benzoate moiety. Fig. 7: Possible mechanism. The oxidative addition of in situ formed Rh(I) catalyst with 4b gives 10 . Subsequent reductive elimination forms optically active biaryl intermediate 11 . The second oxidation addition of 11 with acid anhydride 5 gives 12 , which regenerates Rh(I) catalyst and compound 6 via reductive elimination, followed by hydrolysis. Full size image In conclusion, we reported a Rh-catalyzed asymmetric ring-opening acylation reaction for the synthesis of α-silyl biaryl atropisomers, a class of chiral bulky silanols. The torsional strain of five-membered silafluorenes enabled the success of selective cleavage of C(Ar)–Si bond, thus accomplishing an aryl-Narasaka acylation variant. Additional notable merit of this work is the developed sulfonylpiperazine derived phosphoramidite ligands, which showed high stereo-induction in C(Ar)–Si cleavage/ring-opening reaction. Typical procedure for the Rh-catalyzed aryl-Narasaka acylation Under nitrogen atmosphere, to a Schleck tube was added [Rh(CO) 2 Cl] 2 (2.0 mg, 0.005 mmol, 2.5 mol%), L1 (24.5 mg, 0.021 mmol, 10.5 mol%) and dioxane (2 mL) at room temperature and was stirred for 30 min. The solution was transferred via cannula carefully to another Schlenk tube charged with 4a (62 mg, 0.200 mmol, 1.0 equiv), acetic anhydride (28 μL, 0.300 mmol, 1.5 equiv), Na 2 CO 3 (6.4 mg, 0.060 mmol, 30 mol%), and dioxane (2 mL). 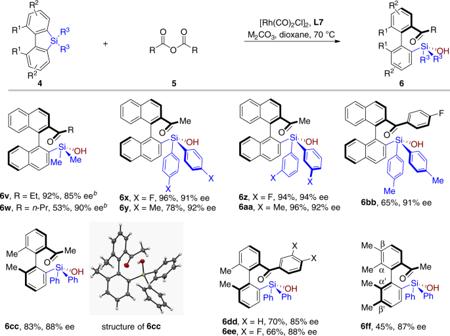Fig. 4: Substrate scopea. aReaction conditions: silafluorene4(0.20 mmol) and acid anhydride5(0.30 mmol, 1.5 equiv), [Rh(CO)2Cl]2(0.005 mmol, 2.5 mol%),L7(0.021 mmol, 10.5 mol%) and base (30 mol%, Na2CO3for aliphatic anhydride, Cs2CO3for aromatic anhydride) in 1,4-dioxane (4.0 mL) at 70 °C for 24 h.bThe reaction was performed withL1as the ligand at 50 °C for 48 h. 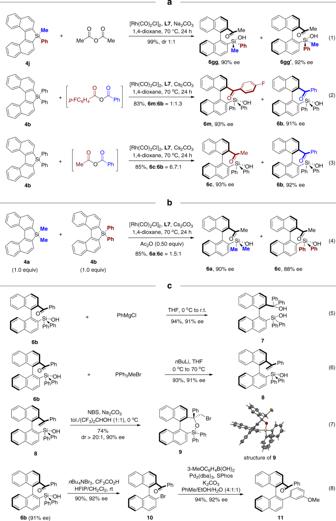Fig. 5: Selectivity for unsymmetrical substrates and synthetic applications. aReactions of nonsymmetric substrates.bReactivity of different substituted substrates using acetic anhydride as limiting reagent.cSynthetic application of axially chiral silanols. 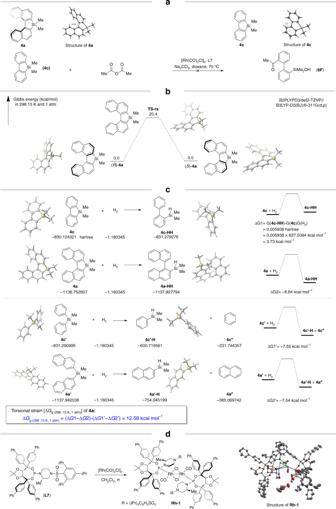Fig. 6: Structure and activity relationship. aRelationship between structure and reactivity of silafluorene.bcalculated rotational barrier energy of4a.cCalculated torsional strain energy of4a.dPreparation of Rhodium-ligand complex. 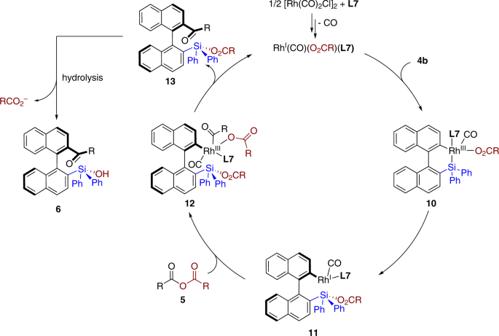Fig. 7: Possible mechanism. The oxidative addition of in situ formed Rh(I) catalyst with4bgives10. Subsequent reductive elimination forms optically active biaryl intermediate11. The second oxidation addition of11with acid anhydride5gives12, which regenerates Rh(I) catalyst and compound6via reductive elimination, followed by hydrolysis. The tube was capped with a screw cap and stirred at 70 °C for 24 h. After being cooled to room temperature, the mixture was filtered through Celite and the filtrate was concentrated in vacuum and purified by flash column chromatography (PE/EtOAc 90:10) on silica gel to afford 6a (73 mg, 98%, 90% ee). \([{\upalpha}]_D^{20}\) −2.25 (c 1.13, CH 2 Cl 2 ). HPLC conditions: Chiralcel AD-H, isopropanol/hexane = 10:90, flow: 1.0 mL/min, λ = 254 nm. 1 H NMR (500 MHz, CDCl 3 ) δ 8.04 (d, J = 9.0 Hz, 1H), 7.99 (d, J = 8.0 Hz, 1H), 7.94 (d, J = 8.5 Hz, 1H), 7.92 (d, J = 8.5 Hz, 1H), 7.87 (d, J = 8.0 Hz, 1H), 7.80 (d, J = 9.0 Hz, 1H), 7.55–7.50 (m, 1H), 7.49–7.44 (m, 1H), 7.31–7.26 (m, 1H), 7.26–7.22 (m, 1H), 7.17 (d, J = 8.5 Hz, 1H), 7.13 (d, J = 8.5 Hz, 1H), 2.70 (s, 1H), 1.94 (s, 3H), 0.13 (s, 3H), −0.47 (s, 3H). 13 C NMR (126 MHz, CDCl 3 ) δ 205.2, 141.5, 138.3, 137.9, 137.4, 134.2, 133.7, 133.5, 132.7, 130.4, 128.7, 128.2, 128.0, 127.6, 127.5, 127.0, 126.6, 126.5, 126.2, 123.9, 30.5, 0.6. HRMS (ESI) calcd for C 24 H 22 O 2 SiNa [M + Na] + 393.1287, found 393.1288.